Circuit reactivation dynamically regulates synaptic plasticity in neocortex Circuit reactivations involve a stereotyped sequence of neuronal firing and have been behaviourally linked to memory consolidation. Here we use multiphoton imaging and patch-clamp recording, and observe sparse and stereotyped circuit reactivations that correspond to UP states within active neurons. To evaluate the effect of the circuit on synaptic plasticity, we trigger a single spike-timing-dependent plasticity (STDP) pairing once per circuit reactivation. The pairings reliably fall within a particular epoch of the circuit sequence and result in long-term potentiation. During reactivation, the amplitude of plasticity significantly correlates with the preceding 20–25 ms of membrane depolarization rather than the depolarization at the time of pairing. This circuit-dependent plasticity provides a natural constraint on synaptic potentiation, regulating the inherent instability of STDP in an assembly phase-sequence model. Subthreshold voltage during endogenous circuit reactivations provides a critical informative context for plasticity and facilitates the stable consolidation of a spatiotemporal sequence. A comprehensive theory of learning and memory requires an understanding of how circuit activity regulates synaptic strength. Hebb [1] postulated that cell assemblies, which are groups of cells that are synaptically linked by repeated co-activation, form a basic computational unit of cortical processing. One cell assembly could instigate activity in another, forming a chain of activations called a phase sequence. Theoretically, phase sequences gain their spatiotemporal structure from the particular pattern and weights of synaptic connections among a population of neurons. The basis of this structure arises from the selective strengthening or weakening of synapses within a circuit. Consistent with Hebb’s postulate, patterns of circuit activity that occur during behaviour recur spontaneously, leading to the hypothesis that the replay of these patterns promotes the synaptic weight changes necessary for learning and memory [2] , [3] , [4] , [5] , [6] , [7] . At the synaptic level, the connection strength between two monosynaptically connected neurons can be experimentally modified by varying the relative time that they fire action potentials [8] , [9] , [10] , [11] , [12] . These spike-timing-dependent plasticity (STDP) protocols are in agreement with Hebb’s hypothesis and suggest a link between studies conducted at the systems level and those made at the level of the single synapse. However, in contrast to classic experimental induction protocols, in vivo recordings show that reactivation of any one pattern of neuronal spikes is sparse and intermittent [2] , [4] , [5] . Recent work has demonstrated that slow-wave activity (SWA), which comprises UP and DOWN states, promotes long term potentiation (LTP), consistent with a role for SWA in memory consolidation [13] , [14] . However, linking endogenously generated spatiotemporal sequences and synaptic plasticity remains largely unexplored. It is particularly important to understand how the temporal contextualization of a synaptic input by an ongoing circuit reactivation determines the plasticity of that input. We set out to test how a temporally structured spontaneous circuit reactivation and the accompanying UP state activity within individual neurons [6] , [15] , [16] , [17] , [18] have an impact on STDP. We use mouse somatosensory thalamocortical slices bulk loaded with the calcium indicator dye Fura 2-AM [19] , to image cortical circuit activity with single-cell resolution. We conduct imaging in combination with patch-clamp recording and observe sparse and intermittent spontaneous UP states during circuit activity. Circuit reactivations showed stereotyped spatiotemporal patterns of neuronal activity, consistent with observations of replay in vivo . To explore the relationship between circuit reactivation and synaptic plasticity, we perform a circuit-dependent pairing protocol. For each pairing, we associate an evoked excitatory synaptic potential with a subsequent brief suprathreshold current pulse in the postsynaptic neuron once per UP state. Imaging reveals that each pairing reliably fell within the same epoch of the circuit sequence during each reactivation. Using this approach, we induce LTP with as few as nine pairings. We find that LTP was dependent on being coincident with the ongoing circuit activity and we term this as circuit-dependent plasticity (CDP). In addition, we find a significant correlation between membrane depolarization during the 20–25 ms interval preceding the pairing and LTP, an effect distinct from the traditional STDP temporal window. Using a spiking neuron network model that exhibits probabilistic sequential recruitment of assemblies, we show that this novel temporal component increases the stable and efficient propagation of a phase sequence while simultaneously shrinking the size, defined by the overall synaptic weight necessary to ensure reliable propagation, of each assembly. Decreasing the synaptic footprint of the assembly is beneficial to maximizing the storage capacity in a neuronal population of fixed number [20] . These data complement previous modelling studies that have shown that spatiotemporal sequences support predictive coding [21] , [22] . Finally, in contrast to STDP, this novel temporal component provides a natural constraint on the strength of a synapse. The naturally occurring stabilization of synaptic strength indicates that the dependence of plasticity on the depolarization within this interval of time acts to prevent the runaway excitation produced by STDP alone. These results suggest an interdependence of memory consolidation and predictive dynamics in the neocortex. Patterned circuit reactivations recur spontaneously All numerical data below are presented as mean±s.d. We targeted layer (L) 2/3 pyramidal neurons for patch-clamp recording in thalamocortical slices of mouse barrel cortex. In the absence of any ionic or pharmacological manipulation, we observed UP states, or spontaneous neuronal activity characterized by periods of prolonged membrane depolarization, during continuous intracellular recording ( Fig. 1a ; 7.5±3.6 mV from rest; 4.16±2.34 s; n =100 UP states; n =8 neurons). UP states occurred in temporally sparse and intermittent intervals (0.022±0.031 Hz; n =93 intervals; n =8 neurons). A power increase in δ -frequency as measured in the membrane voltage recordings of patch-clamped neurons accompanied the transition to the UP state (16.1±12.7-fold; n =100 UP states; n =8 neurons). We tracked spiking activity within the surrounding neuronal population using multiphoton laser-scanning microscopy of neurons loaded with the calcium indicator dye Fura-2AM [23] , [24] . Spike trains were inferred from somatic fluorescence measures [23] , [24] . Imaging conducted simultaneously with patch-clamp recordings demonstrated that a population-level neuronal firing was coincident with a single-cell depolarization ( Fig. 1a,b,c ). Thus, the UP state is the neuronal substrate for circuit activity [15] , [16] , [17] , [25] , [26] . We refer to the recurrence of these distinct spontaneous events as circuit reactivations. 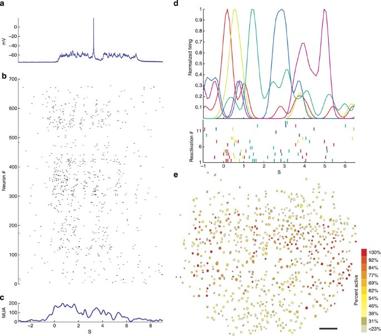Figure 1: Recurrence of UP states and circuit activity is characterized by stereotyped spatiotemporal sequences within the imaged population. (a–c) An example of a spontaneous circuit reactivation, indicating both the accompanying single-cell depolarization and the detected action potentials within the field of view. Physiology and raster are aligned in time. (a) A single-cell UP state in a patch-clamped L2/3 pyramidal neuron during a circuit reactivation. The action potential is truncated for display purposes. (b) Raster plot of detected action potentials from fluorescence imaging during the same circuit reactivation. (c) Multi-unit average (MUA), indicating population firing rate over time. (d) Ca2+imaging reveals temporal structure of circuit reactivations. Lower panel: spike times of five stereotyped neurons are indicated in raster. Upper panel: convolved spike times over 13 reactivations. (e) Spatial location of active neurons. Colour code indicates reliability of activity over the 13 trials corresponding tob. Scale bar, 100 μm. Figure 1: Recurrence of UP states and circuit activity is characterized by stereotyped spatiotemporal sequences within the imaged population. ( a – c ) An example of a spontaneous circuit reactivation, indicating both the accompanying single-cell depolarization and the detected action potentials within the field of view. Physiology and raster are aligned in time. ( a ) A single-cell UP state in a patch-clamped L2/3 pyramidal neuron during a circuit reactivation. The action potential is truncated for display purposes. ( b ) Raster plot of detected action potentials from fluorescence imaging during the same circuit reactivation. ( c ) Multi-unit average (MUA), indicating population firing rate over time. ( d ) Ca 2+ imaging reveals temporal structure of circuit reactivations. Lower panel: spike times of five stereotyped neurons are indicated in raster. Upper panel: convolved spike times over 13 reactivations. ( e ) Spatial location of active neurons. Colour code indicates reliability of activity over the 13 trials corresponding to b . Scale bar, 100 μm. Full size image Continuous rapid imaging of circuit reactivations using a heuristically optimized path scan [23] allowed us to identify temporally precise and reliable neuronal firing sequences within the circuit ( Figs 1d,e and 2 ). We compared imaged circuit reactivations using a cost-based metric, where increasing dissimilarity between circuit reactivation spike patterns is associated with an increased cost [27] ( Fig. 2a ). A measure of the similarity between spike trains within the same neuron across multiple circuit reactivations was used to generate a measure of spike-time precision for that neuron. We calculated the distance between each spike train within an individual neuron that we termed characteristic distance ( Fig. 2b ; see Methods). Using this measure, we established statistical significance of neuronal spike-time stereotypy by comparing the experimentally measured spike times with spike times resampled from an inhomogeneous Poisson distribution defined by the population firing rate ( Figs 1c and 2b,c ; see Methods). An additional test was performed by testing against shuffled spike trains (see Methods) and neurons were only considered stereotyped if they were significant for both tests. We found that 28.5% of neurons were significantly precise in time over multiple trials ( Figs 1d and 2d ). These stereotyped circuit reactivations provided us with an experimental model for the study of synaptic plasticity in a naturalistic and circuit-dependent context. 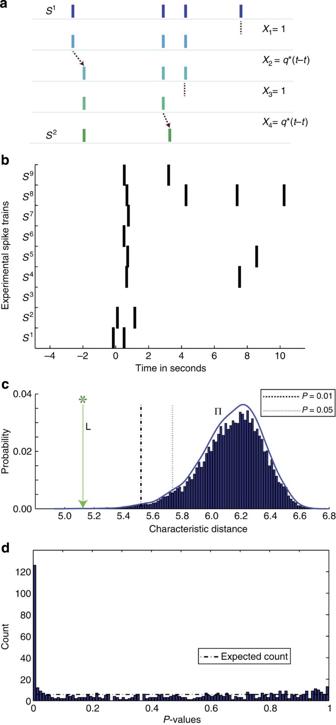Figure 2: Identification of temporally stereotyped cells detected using multiphoton laser-scanning microscopy. (a) An example of how two spike trainsandare compared by a sum of costs in equation (1). EachXiis the cost of a single transition where a spike is removed, added or shifted to transformto. (b) An example of a significantly stereotyped cell. Raster plot indicates inferred action potentials over different circuit reactivations for which distance has been calculated. (c) The characteristic distance, equation (2), between all of a neuron’s spike trainsacross all circuit reactivations (green arrow labelled L) is compared against the distribution of characteristic distances (labelledπ) of the null spike trains (histogram and smoothed curve)n=9 circuit reactivations. This cell was significantly stereotyped (asterisk) as compared with reshuffled data (binomial test,P<0.05,n=10,000 trials; see Methods). (d) The distribution ofP-values for temporal stereotypy across all neurons. Values are from the experiment inFig. 1. Many more neurons are stereotyped then would be expected from chance levels, although another set of neurons do not show a clear degree of temporal stereotypy. Figure 2: Identification of temporally stereotyped cells detected using multiphoton laser-scanning microscopy. ( a ) An example of how two spike trains and are compared by a sum of costs in equation (1) . Each X i is the cost of a single transition where a spike is removed, added or shifted to transform to . ( b ) An example of a significantly stereotyped cell. Raster plot indicates inferred action potentials over different circuit reactivations for which distance has been calculated. ( c ) The characteristic distance, equation (2) , between all of a neuron’s spike trains across all circuit reactivations (green arrow labelled L) is compared against the distribution of characteristic distances (labelled π ) of the null spike trains (histogram and smoothed curve) n =9 circuit reactivations. This cell was significantly stereotyped (asterisk) as compared with reshuffled data (binomial test, P <0.05, n =10,000 trials; see Methods). ( d ) The distribution of P -values for temporal stereotypy across all neurons. Values are from the experiment in Fig. 1 . Many more neurons are stereotyped then would be expected from chance levels, although another set of neurons do not show a clear degree of temporal stereotypy. Full size image Reliable recruitment of functionally assembled units Within a Hebbian framework, we postulated interdependence between circuit reactivations and synaptic plasticity. To test this hypothesis, it was necessary to reliably control a temporal segment of the circuit reactivation. We evoked a functional assembly of neurons using minimal extracellular stimulation ( Fig. 3a ). To be considered a functionally assembled unit, the same small number of neurons had to be consistently recruited and have a stable output onto a postsynaptic ‘reader’ neuron [7] . Imaging of the area surrounding the stimulating electrode in L4 revealed that a small population of neurons were reliably activated (0.6±0.9 neurons active in a single imaging plane over 80% of the time; n =5 stimulator placements; Fig. 3b , red neurons). We detected the postsynaptic effect of these stimulated sets of neurons as compound excitatory post synaptic potentials (EPSP)s, recorded during the DOWN state, within individual circuit L2/3 pyramidal neurons ( Fig. 3b , inset). Consistent with the imaging data, we found a patch-clamp recorded compound EPSPs to have reliable and stable amplitudes (2.4±1.5 mV, n =20; Fig. 3c ). We evaluated the stability of the measured EPSP amplitudes using bootstrap reshuffling ( Fig. 3d ). These data demonstrate that we consistently and reliably activated a set of neurons, or a functional assembled unit, and ‘read’ its output within individual L2/3 neurons. 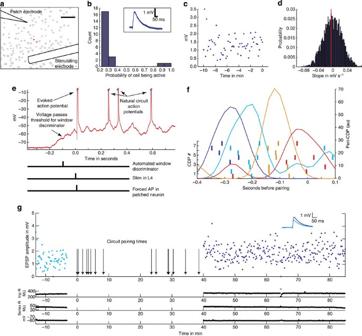Figure 3: STDP during circuit reactivation results in LTP. (a) A small reliable population of neurons responded to the stimulating electrode. Red cells responded at least 80% of the time. Scale bar, 50 μm. (b) Histogram of the probability that any neuron within the imaged field will respond to the applied stimulus from the same experiment ina. Only cells that fired in response to more than one stimulation are included. (c) The average EPSP recorded in a L2/3 pyramidal neuron across all stimulations from the same experiment. Ten minutes of EPSP amplitudes were tested for stability before pairing. (d) The distribution of EPSP amplitude drift after bootstrap reshuffling the residuals to the best linear fit. The red line indicates the slope with no shuffling. (e) Online detection of a circuit reactivation was accomplished using a window discriminator triggered off of the accompanying membrane depolarization in the patched L2/3 cell. After a fixed delay, a circuit pairing was activated. Action potentials are truncated for display purposes. (f) Ca2+imaging reveals that temporal structure of the circuit reactivation is preserved when aligned relative to the time of the circuit pairing (t=0). Raster plots of cells for multiple circuit pairings (leftyaxis), where colour indicates cell identity, show preservation in the order of firing between neurons. Superimposed are response curves of these same cells (right axis). All responses are aligned to the pairing. (g) Example of a CDP experiment. Baseline individual EPSP amplitudes are illustrated (light blue). Circuit pairings were executed based on online detection of spontaneous circuit reactivations (black arrows) over the time course of 40 min. After circuit pairings, individual EPSP amplitudes are illustrated (dark blue). Inset: the average EPSP amplitude before (n=60, light blue) and after circuit pairing (n=60, dark blue). Input resistance, series resistance and resting membrane potential were all monitored for stability during the testing of EPSPs. The asterisk represents a spontaneous circuit reactivation during the test period, transiently shifting the measures. Figure 3: STDP during circuit reactivation results in LTP. ( a ) A small reliable population of neurons responded to the stimulating electrode. Red cells responded at least 80% of the time. Scale bar, 50 μm. ( b ) Histogram of the probability that any neuron within the imaged field will respond to the applied stimulus from the same experiment in a . Only cells that fired in response to more than one stimulation are included. ( c ) The average EPSP recorded in a L2/3 pyramidal neuron across all stimulations from the same experiment. Ten minutes of EPSP amplitudes were tested for stability before pairing. ( d ) The distribution of EPSP amplitude drift after bootstrap reshuffling the residuals to the best linear fit. The red line indicates the slope with no shuffling. ( e ) Online detection of a circuit reactivation was accomplished using a window discriminator triggered off of the accompanying membrane depolarization in the patched L2/3 cell. After a fixed delay, a circuit pairing was activated. Action potentials are truncated for display purposes. ( f ) Ca 2+ imaging reveals that temporal structure of the circuit reactivation is preserved when aligned relative to the time of the circuit pairing ( t =0). Raster plots of cells for multiple circuit pairings (left y axis), where colour indicates cell identity, show preservation in the order of firing between neurons. Superimposed are response curves of these same cells (right axis). All responses are aligned to the pairing. ( g ) Example of a CDP experiment. Baseline individual EPSP amplitudes are illustrated (light blue). Circuit pairings were executed based on online detection of spontaneous circuit reactivations (black arrows) over the time course of 40 min. After circuit pairings, individual EPSP amplitudes are illustrated (dark blue). Inset: the average EPSP amplitude before ( n =60, light blue) and after circuit pairing ( n =60, dark blue). Input resistance, series resistance and resting membrane potential were all monitored for stability during the testing of EPSPs. The asterisk represents a spontaneous circuit reactivation during the test period, transiently shifting the measures. Full size image Circuit activity facilitates LTP To explore the relationship between circuit reactivation and synaptic plasticity, we associated a synaptic input and an evoked action potential once per UP state ( Fig. 3e ). We achieved this by extracellular stimulation in L4, as described above, followed by the application of a brief suprathreshold intracellular current pulse in the patch-clamped postsynaptic neuron (see Methods). Online monitoring of the membrane depolarization within circuit neurons (LabView) allowed us to detect the ongoing circuit activity and to activate our pairing once per UP state ( Fig. 3e ). Multiphoton imaging indicated that by using this approach, the timing of the circuit pairing reliably fell within a particular epoch of the temporal circuit pattern ( Fig. 3f ). We evaluated the impact of endogenous circuit reactivation and the accompanying neuronal depolarization on the emergence of LTP. Within 35–45 min, we applied as few as 9 and as many as 29 circuit pairings (17.88±6.90, n =8 neurons). The number of circuit pairings varied across data sets, as there was no fixed interval between circuit reactivations. The average frequency of occurrence of circuit pairings was low (interval duration 105.68±124.24 s; n =8 neurons). After the circuit-pairing period, we again measured the evoked EPSP amplitude during the DOWN state. We found significant increases in the amplitude of the EPSPs (116.1%±19.1% of baseline mean±s.d. ; n =8 neurons, P =0.048; Fig. 3f ). Thus, despite these sparse and intermittent protocols, and the presence of intact inhibition, we induced LTP. Previous experiments have demonstrated that pairing interval(s) and intracellular depolarization are key metrics for the emergence of LTP [10] , [11] . As a result, we ran two sets of controls. First, to address the intermittent circuit pairing intervals in the experiment, we customized every single control using interval-matched pairings identical to that of the CDP trials and also ensured that a pairing was not associated with a circuit reactivation ( Fig. 4a ). Thus, each interval control had the same number of pairings and identical pairing intervals to a matched CDP experiment. The amplitude of EPSPs after these quiescent pairings were significantly different from CDP pairings (72.8±30.6%, n =6; CDP versus interval control, P =0.007; Fig. 4a ). Second, we customized each control to match the UP state depolarization (8.12±0.94 mV), duration (5.06±0.12 s) and specific intervals using somatic intracellular current injection to each matched CDP experiment ( Fig. 4b ). Again, changes in EPSP strength were significantly different from CDP experiments (amplitude of EPSPs after pairings with experimental depolarization, 71.3±22.8%; n =6; CDP versus depolarization controls, P =0.002; Figs 3 and 4c ). Similar results demonstrating the inability of somatic current injection to promote LTP have been shown in previous studies in L2/3 neurons [28] . Finally, we monitored the amplitude of EPSPs over a prolonged time course (50 min) to control for the fact that these are long protocols. We find that overall there is a trend towards LTD ( n =45; 76.09% change±23.48%; CDP versus no pairings, P =3.24 × 10 −5 ). These data demonstrate that circuit activity is necessary for the induction of LTP using sparse and intermittent induction protocols. 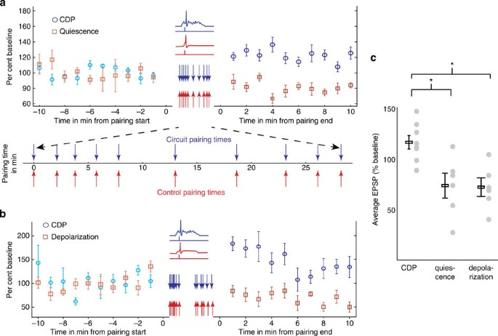Figure 4: Interval-matched quiescent and depolarized controls do not demonstrate LTP. In bothaandb, EPSP amplitudes are illustrated by blue circles (CDP) and red squares (control pairing) representing the mean±s.e.m. EPSP amplitude over 1 min. Inset is a schematic of the respective control pairings (blue for the CDP and red for the Control). In both cases, the top trace represents the L2/3 neuron and bottom trace represents the L4 stimulation. For any given trial, CDP pairing times (blue arrows) are matched when pairing during controls (red arrows). (a) An example of an interval-matched control experiment from quiescence. The time expansion bellow illustrates the matched intervals between the control and experimental conditions. (b) An example of a depolarization and interval-matched control experiment. (c) Pooled results of the per cent change in EPSP amplitude showing each individual data point (grey) and the mean±s.e.m. (black). CDP is compared with interval-matched controls from quiescence and interval-matched controls with depolarization. Asterisks denote significance ofP<0.05, Student’st-test,n=8; CDP experiments,n=6 quiescence controls,n=6 depolarization controls. Figure 4: Interval-matched quiescent and depolarized controls do not demonstrate LTP. In both a and b , EPSP amplitudes are illustrated by blue circles (CDP) and red squares (control pairing) representing the mean±s.e.m. EPSP amplitude over 1 min. Inset is a schematic of the respective control pairings (blue for the CDP and red for the Control). In both cases, the top trace represents the L2/3 neuron and bottom trace represents the L4 stimulation. For any given trial, CDP pairing times (blue arrows) are matched when pairing during controls (red arrows). ( a ) An example of an interval-matched control experiment from quiescence. The time expansion bellow illustrates the matched intervals between the control and experimental conditions. ( b ) An example of a depolarization and interval-matched control experiment. ( c ) Pooled results of the per cent change in EPSP amplitude showing each individual data point (grey) and the mean±s.e.m. (black). CDP is compared with interval-matched controls from quiescence and interval-matched controls with depolarization. Asterisks denote significance of P <0.05, Student’s t -test, n =8; CDP experiments, n =6 quiescence controls, n =6 depolarization controls. Full size image The 20–25 ms preceding the pairing correlates with CDP Depolarization in the postsynaptic neuron has been shown to be a key factor for determining the amplitude of plasticity [11] , [12] , [29] , [30] , [31] , [32] . As a result, we calculated the correlation between depolarization and the measured LTP amplitude. We found that depolarization during a specific epoch of the UP state highly correlated with potentiation. Specifically, we found a peak in Pearson’s correlation of CDP with depolarization during the 20- to 25-ms window preceding the circuit pairing ( Fig. 5a ; r =0.71, P =0.047). To control for the confounding effect of membrane depolarization at other times, we used a partial correlation statistic. To do so, we conditioned the measure of correlation within individual time bins on the depolarization across the 100 ms preceding the pairing. Voltage was stable in mean and variance during this period ( Fig. 5b ). This analysis further sharpened the effective time period ( r =0.897, P =0.0062 for the 20 and 25 ms time bins). In contrast, the correlation immediately preceding the pairing, in the 0- to 5-ms bins, was weak and within chance levels ( r =0.335, P =0.51; Fig. 5a ). The partial correlation analysis was not sensitive to the use of the 100-ms baseline level, as conditioning on 50 ms preceding the pairing yielded similar results ( r =0.88, P =0.009). Similarly, the peak in the correlation between voltage and LTP was independent of the size of the time bin used to calculate the correlation (10 ms bin of 20–30 ms, r =0.87, P =0.011, and using 1 ms bin of 24–25 ms, r =0.90, P =0.0064). This analysis suggests that the temporal structure inherent to the circuit, as manifested in the synaptically driven subthreshold membrane depolarization of individual neurons, determines the amplitude of LTP. Moreover, a period preceding the pairing proved to be highly correlated with the amplitude of LTP. 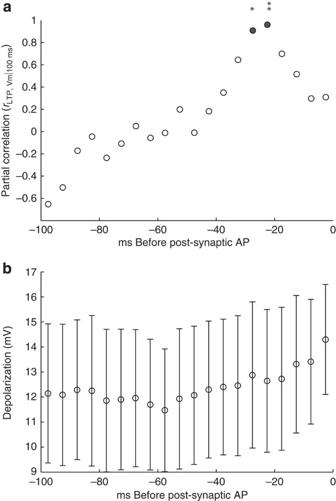Figure 5: Potentiation correlates with UP state depolarization in a time-dependent manner. (a) Partial correlation, equation (5), the correlation of potentiation with median membrane depolarization from rest, binned in 5 ms windows before the injected action potential conditioned on the membrane potential during the preceding 100 ms (see Methods). Grey points indicate significant correlation. *P<0.05, **P<0.01, partial correlation,n=8. (b) The median membrane depolarization from rest binned in 5 ms windows before the L4 stimulation±s.d.,n=8. Voltage did not systematically change across the period immediately preceding the pairing. Figure 5: Potentiation correlates with UP state depolarization in a time-dependent manner. ( a ) Partial correlation, equation (5) , the correlation of potentiation with median membrane depolarization from rest, binned in 5 ms windows before the injected action potential conditioned on the membrane potential during the preceding 100 ms (see Methods). Grey points indicate significant correlation. * P <0.05, ** P <0.01, partial correlation, n =8. ( b ) The median membrane depolarization from rest binned in 5 ms windows before the L4 stimulation±s.d., n =8. Voltage did not systematically change across the period immediately preceding the pairing. Full size image Spiking network model of a Hebbian phase sequence We explored the consequences of CDP in a network model that comprises adapting spiking neurons [34] . We set out to evaluate the effect of the CDP rule, defined as a scaling factor for STDP determined by the membrane voltage 25 ms before a synaptic input (see Methods) on three metrics: (1) the progression of an assembly phase sequence, (2) synaptic potentiation and (3) overall synaptic ‘footprint’ of an assembly. We then compared and contrasted these results with the same metrics in models in which we applied a standard STDP rule. Our model generated a phase sequence described by a probabilistic propagation of activity from one assembly to the next. We constructed phase sequences by starting with a default recurrent network of 1,800 neurons. We then assembled independent subsets of 100 neurons with increased levels of connectivity and synaptic weight. These assemblies were then interconnected, allowing probabilistic transitions between them ( Fig. 6a ). A random transient input (20 ms) into the first assembled population initiated UP states from quiescence. Once the UP state is initiated, depolarization within neurons was dictated by both recurrent connections in the assembly and feed-forward input from the preceding assembly ( Fig. 6a ). The depolarization, in the 25-ms window preceding pairing, determined the amount of potentiation that occurs in the CDP condition (see Methods). 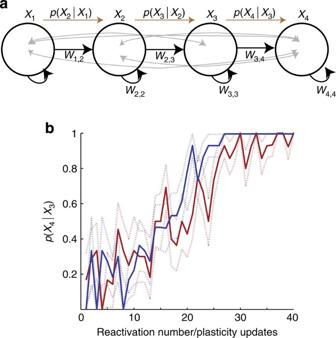Figure 6: Model of an assembly phase sequence with an STDP or a CDP plasticity rule shows progressively more reliable propagation of the sequence. (a) Assemblies,Xi, are represented by the circles and connections between and within them by arrows with weightswi,j. There is an additional default recurrent network, light grey arrows. The model reveals probabilistic propagation between assemblies (gold arrows withp(Xi|Xi−1)). (b) The transition probability fromX3toX4after iterative updates in plasticity of either CDP (blue) or STDP (red). Error bars are s.e.m.,n=15 simulations. Figure 6: Model of an assembly phase sequence with an STDP or a CDP plasticity rule shows progressively more reliable propagation of the sequence. ( a ) Assemblies, X i , are represented by the circles and connections between and within them by arrows with weights w i,j . There is an additional default recurrent network, light grey arrows. The model reveals probabilistic propagation between assemblies (gold arrows with p(X i |X i −1 )). ( b ) The transition probability from X 3 to X 4 after iterative updates in plasticity of either CDP (blue) or STDP (red). Error bars are s.e.m., n =15 simulations. Full size image We first evaluated the impact of CDP and STDP (see Methods) on the propagation of the phase sequence. Both CDP and STDP rules produced increasing likelihood of phase-sequence propagation with each subsequent circuit reactivation. Increasing transition probability indicated more reliable recruitment from one assembly to the next ( Fig. 6b ), eventually leading to completion of the full phase sequence ( Fig. 7 ). The fact that both STDP and CDP resulted in progressive sequence propagation satisfied an important benchmark [35] for the two plasticity rules. We then examined the effect each rule had on synaptic weights in the model. The multiplicative STDP rule caused weights to increase rapidly and without being bound with successive reactivations ( Fig. 8a ). In contrast, the CDP rule increased synaptic strength up to a stable value despite continued reactivations ( Fig. 8a ). Consistent with a putative role for CDP in memory consolidation, CDP also caused a subset of the synaptic weights to decrease to a value of zero. This in turn resulted in a decrease in the mean synaptic weight within an assembly while maintaining a reliable assembly phase sequence ( Fig. 8b ). STDP initially produced a decrease in the overall synaptic weights; however, this decrease was transient and weights did not stabilize ( Fig. 8b ). How does CDP stabilize potentiation? In the model, a postsynaptic neuron only received high levels of depolarization if it fired slightly later then its assembled counterparts. With successive reactivations and the resultant LTP, it achieved threshold earlier. As a result, because postsynaptic firing time moved closer to circuit-generated peaks in its subthreshold potential, it escaped the CDP window. For that postsynaptic neuron, LTP led to earlier firing, effectively decreasing the preceding depolarization and limiting additional LTP. These results demonstrate that the CDP rule ensures stable propagation of an assembly phase sequence, while minimizing the size of an assembly. In addition, CDP drives the strongest synaptic weights to an asymptotic level over successive reactivations that stabilize the model. 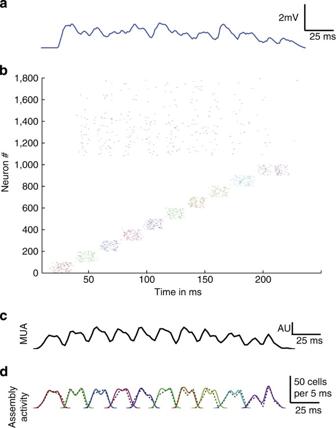Figure 7: An example of a full assembly phase sequence involving ten assemblies after multiple plasticity updates. All figure parts are aligned in time (a). An example of subthreshold activity during the assembly as seen in a cell not assigned to an assembly. (b) The spike raster activity during the phase sequence. Black ticks indicate inhibitory neuronal spiking. Coloured ticks are from the population of excitatory neurons, where each assembly is labelled with a different colour. (c) The multi-unit average, indicating population firing rate. (d) Isolated activity of individual assemblies. Each colour corresponds to a different assembly as ina. Bold coloured lines represent the smoothed spiking activity. Black dotted lines represent the spiking activity in 5 ms bins. Figure 7: An example of a full assembly phase sequence involving ten assemblies after multiple plasticity updates. All figure parts are aligned in time ( a ). An example of subthreshold activity during the assembly as seen in a cell not assigned to an assembly. ( b ) The spike raster activity during the phase sequence. Black ticks indicate inhibitory neuronal spiking. Coloured ticks are from the population of excitatory neurons, where each assembly is labelled with a different colour. ( c ) The multi-unit average, indicating population firing rate. ( d ) Isolated activity of individual assemblies. Each colour corresponds to a different assembly as in a . Bold coloured lines represent the smoothed spiking activity. Black dotted lines represent the spiking activity in 5 ms bins. 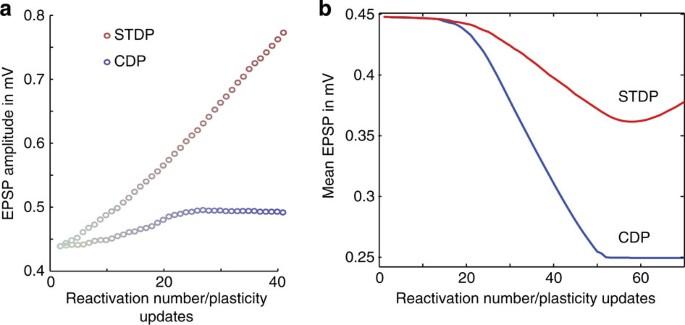Figure 8: CDP stabilizes LTP and shrinks the synaptic footprint of an assembly. (a) An example illustrating the progression of potentiated weights for a single synapse in assemblyX3after successive applications of the STDP (red) or CDP (blue) rule corresponding to the number of reactivations. Shading is a visual aid with darker colours having further plasticity updates. (b) The mean of the full distribution of synaptic weights for assemblyX3over successive applications of a plasticity rule STDP (red) and for CDP (blue). Full size image Figure 8: CDP stabilizes LTP and shrinks the synaptic footprint of an assembly. ( a ) An example illustrating the progression of potentiated weights for a single synapse in assembly X 3 after successive applications of the STDP (red) or CDP (blue) rule corresponding to the number of reactivations. Shading is a visual aid with darker colours having further plasticity updates. ( b ) The mean of the full distribution of synaptic weights for assembly X 3 over successive applications of a plasticity rule STDP (red) and for CDP (blue). Full size image There is evidence to support the theory that memories are rapidly formed in the hippocampus during behaviour and transferred to the neocortex during slow-wave sleep for long-term storage [36] , [37] . Repeating sequences during SWA and quiet wakefulness have been shown to reflect previous sensory experience [2] , [7] . Interruption of replay [14] obstructs behavioural recollection of learned tasks. As a result, repetition of sequences may have an important role in learning and memory consolidation [2] , [4] , [5] , [7] . This has been convincingly demonstrated in the juvenile songbird system, where specific replay of neuronal activity during sleep resulted in appropriate changes in the bird’s song the following day [3] . The importance of reactivation to memory is clear from these systems-level studies. Circuit reactivation in slice is remarkably similar to activity in vivo during SWA [25] , [26] and provides a useful tool to examine synaptic plasticity in this context [13] . We find that circuit reactivations in vitro display stereotyped spatiotemporal patterns of neuronal activity consistent with observations of replay in vivo . In addition, we confirm that reactivation is synonymous with subthreshold depolarized UP states in individual neurons. Postsynaptic depolarization is a key determinant for the emergence of LTP [11] , [12] , [29] , [30] , [31] , [32] . However, it remains unclear whether endogenous circuit activity was capable of potentiating an associated synaptic input if each recurrence of an association was sparse and intermittent. Furthermore, it is unclear how the contextualization of a synaptic input by the temporal structure inherent to memory trace replay would impact synaptic plasticity. Our data addresses these questions directly. We show here that endogenously arising UP states facilitate the emergence of LTP following a few sparse and intermittent pairings coincident with ongoing circuit reactivation. This is consistent with data showing that multiple synaptic inputs have a cooperative effect on the induction of LTP [11] , [38] . Similarly, the UP state is the byproduct of multiple synaptic inputs and it is likely that these inputs act cooperatively. We note in our experiments that although the net result of the synaptic drive is the depolarization that defines the UP state, the endogenously arising synaptic drive is composed of both inhibitory and excitatory synaptic inputs [33] , indicating that naturalistic circuit activity supports LTP despite intact inhibition. Our experimental results add feasibility to the postulate that the replay of sequential circuit activity in vivo is capable of strengthening synaptic connections, complementing previous work demonstrating that STDP can be evoked in the intact organism [39] , [40] . Our experiments indicate that the UP state is not a single unit over which plasticity of a single synaptic input is integrated. Rather, the depolarization during the 20- to 25-ms interval preceding the pairing most highly and significantly correlates with the observed CDP in contrast to the depolarization at the time of pairing. This result is very similar to a hippocampal study that reports input timing-dependent plasticity. In that investigation, distal input from the perforant path induces plasticity of Schaffer collateral input through an NMDA ( N -methyl- D -aspartate)-receptor-mediated mechanism when the two were separated by an appropriate interval [41] . This suggests two possibilities to explain our results. First, that distal dendritic inputs onto the patch-clamped L2/3 pyramidal neuron act as an instructive signal for the LTP of L4 inputs via the NMDA receptor activation [41] . These data would suggest that single-cell properties dictate which temporal features of the circuit-dependent synaptic drive are linked together through synaptic plasticity. Alternatively, there may be a relevant timescale of circuit dynamics for synaptic plasticity [42] that may reflect aspects of sensory input [43] , consistent with the Hebbian phase-sequence hypothesis [1] . Together, these two possibilities would imply that circuit dynamics and their relevant timescales are emergent from both single-cell and circuit-dependent synaptic properties. In predictive models of spike timing, similar intervals have been shown to have the greatest efficacy when considering spikes from co-active neurons [7] , [44] . Recent reports have described the clustering of synaptic inputs on a dendritic arbour during spontaneous activity [45] , [46] , [47] that may result in a cooperative amplification between spines [48] . The temporal relationship and specific locus of the synaptic input are probably the key to determining whether an input or set of inputs is potentiated [41] , [42] , [49] . It may be that the temporal structure of the circuit results in stereotyped activation of dendritic arbours that determines plasticity of associated synapses. Synaptic plasticity involves the selective strengthening or weakening of synapses necessary for learning and memory. Reinforcement of relevant synapses results in the reliable flow of information or propagation of activity from one circuit to the next [50] and is thought to promote memory consolidation. Other theories of consolidation have emphasized global synaptic depression in conjunction with sparser potentiation, resulting in system-wide synaptic homeostasis [51] . Consistent with these theories, our results show LTD in synapses, which are not associated with CDP. Further, our modelling studies illustrate a net decrease in synaptic weights when considering CDP in the context of a phase sequence ( Fig. 8b ). Our model of an assembly phase sequence shows that with repeated activation, both STDP and CDP rules result in the reliable propagation of a phase sequence. This is consistent with previous work that has shown that STDP rules support the emergence of predictive dynamics [21] , [22] . We find that CDP rules stably shrink the footprint of any one assembly within the synaptic weight matrix. Assuming a fixed number of neurons, shrinking the size of the assembly will increase the number of possible assembly phase sequences and the storage capacity of the system [20] , [50] , [52] which may be an important aspect of memory consolidation. Multiplicative STDP has long been known to be inherently unstable [53] , [54] , except in the cases when synaptic strengths are explicitly bounded [55] , [56] or in cases when functionally similar constraints are imposed [53] , [54] , [57] . In the bounded STDP case, plasticity effectively pushes the circuit towards a binary regime of saturated or silent synapses. We find that CDP naturally regulates the amplitude of synapses forcing these strengths to an asymptotic level without the requirement of explicitly setting a bound on synaptic strength. The fact that CDP stabilizes synaptic weights, rather than saturating them, leaves the potential to preserve flexibility through dynamic gradation of synaptic strength. We speculate that this stabilization results from the dynamic interaction between the timing of the phase sequence and CDP, creating a temporally regulated negative feedback mechanism for LTP. Slice preparation Thalamocortical slices, 450-μm thick, were prepared from postnatal day 15 (P15) to P19 C57BL/6 mice of both genders with a vibratome (VT1000S) [16] , [58] . Mice were anaesthetized by intraperitoneal injection of ketamine–xylazine. All procedures were approved by the Institutional Animal Care and Use Committee at the University of Chicago. Electrophysiology and two-photon imaging Whole-cell voltage-clamp and current-clamp recordings were carried out using Multiclamp 700B amplifiers (Axon Instruments, Foster City, CA). Custom-built software (Labview) was used for controlling Multiclamp and stimulation electrodes via a DAQ board (6733; National Instruments). Electrophysiological signals from whole-cell patch recordings were digitized at 10 kHz. Recordings were performed at room temperature in standard artificial cerebral spinal fluid containing (in mM) 123 NaCl, 3 KCl, 26 NaHCO 3 , 1 NaH 2 PO 4 , 2 CaCl 2 , 2 MgSO 4 and 25 dextrose, which was continuously aerated with 95% O 2 and 5% CO 2 . Patch pipettes 5–11 MΩ were filled with (in mM) 135 K -gluconate, 8 KCl, 10 HEPES, 4 ATP-Mg, 0.3 GTP-Tris and 10 Na 2 -Phosphocreatine (pH 7.2, 290–295 mOsm), and occasionally biocytin and/or Alexa 488 (20 μM). Imaging data were acquired with a custom-built multiphoton microscope, using a femtosecond-pulsed Chameleon Ultra II Ti:sapphire laser (Coherent; λ =790 nm). To maximize the speed of fluorescence measures from large populations of neurons using a standard multiphoton laser-scanning microscopy setup, we employed Heuristically Optimal Path Scanning, which provides user parameter-controlled and computationally optimized scans of many targets and allowed us to optically monitor a population of neurons in a field of view at high rates with a single spike resolution [23] . Online and offline image analyses were carried out using custom-written software (MATLAB, Python). The most probable spike train was then modelled from Fura-2AM fluorescence changes [23] , [24] . Analysis of temporal structure in circuit reactivations We established statistical significance of temporal stereotypy for each cell in a field of view by comparing all the individual spike trains of a cell obtained from every circuit event. We represent a spike train as an ordered set of s spike times for any cell i during a circuit reactivation l . If a cell did not participate in at least five circuit reactivations, it was not used in any analyses for temporal structure. To assess the temporal similarity between two spike trains, , , we use a cost-based metric, (refs 27 , 59 ), which formulates a distance between two spike trains accounting for the number of spikes in each train and the timing between them parameterized by a temporal component q . We define the distance between two spike trains by a set of transformations needed to make the spike trains equal in their spike times with a minimal cost, where is the set of transformations, which turn into , and the function establishes the cost of those transformations ( Fig. 2a ). We compute the overall similarity of a neuron firing across circuit reactivations. We define the characteristic distance L , by looking at all pairs of spike-time distances from different circuit reactivations and taking the mean ( Fig. 2c , arrow). To establish whether a characteristic cost is significant given the spike trains observed, we define a null distribution over L i . We generate null spike trains where the number of spikes are the same as in . We do this by finding the population firing rate λ ( t ) and normalizing this into a PDF λ *( t ). Next, we draw from λ *( t ) matching the number of spikes in a given spike train. We define λ ( t ) such that it reflects the level of overall network activity separately for each circuit reactivation λ l ( t ), accounting for intertrial variability of circuit reactivations ( Fig. 1c ). A new with different are calculated 10,000 times to form a distribution of expected given the neurons’ number of spikes, and the time course of activity as in equation (2). The neurons’ temporal similarity, L i , is then compared with this distribution of to form a probability value against this null hypothesis p Poission . Neurons were considered to be significantly stereotyped by the binomial test (binofit.m; MATLAB). To test that our results are robust, we used a second null hypothesis that avoids the use of Poisson-generated spike trains. We shuffle spike trains by changing the spike train’s neuron identity, while maintaining its circuit reactivation identity, we use random permutations of to generate and define a distribution of to compare against L i and obtain a second assessment of P -value, p Shuffle . Permutations across were performed only against spike trains with the same number of spikes. Analysis of extracellularly activated neurons Evoked sets of neurons were activated using an extracellular bipolar electrode (platinum iridium CE2C55, Frederick Haer Co., Bowdoinham, ME) to inject brief, 1-ms current pulses (Iso-flex stimulator, AMPI, Jerusalem, Israel) of a minimal amplitude (mean 9.73±8.56 μA) [30] . Resultant EPSPs were recorded in the current clamp and analysed for their peak amplitude in MATLAB. In bulk-loaded slices, functional assemblies were imaged around the stimulating electrode [60] . Cells that were reliably active in at least 80% of trials were considered reliable ( Fig. 3a,b ). Plasticity protocols Online detection of circuit reactivations was achieved using a software-based window discriminator that monitored the membrane potential of a patch-clamped neuron (Labview). We triggered a circuit pairing whenever a cell reached a threshold between 7 and 15 mV from rest. Circuit pairings occurred between 100 and 200 ms after the detection of neuronal depolarization. The pairing comprises an EPSP that was evoked by using extracellular stimulation in L4 followed by a 5-ms depolarizing 813±270-pA pulse injected via the patch pipette, which was sufficient to force an action potential in the postsynaptic neuron. Note that the UP state is a high-conductance condition [17] . The lag between the evoked EPSP and the evoked spike was 10 ms. For control pairings, intervals were tracked online (Labview). For depolarization controls, current pulses were injected into the cell to approximate the median depolarization of UP states, and circuit pairings were performed 100–200 ms after the start of depolarization. For post-hoc analysis, UP states were detected in one of the two ways: (1) a period of boxcar-average of more than 5 mV above the baseline for at least 500 ms or (2) a period of boxcar-average that is more than 3 mV above baseline and firing rate was at least 6 Hz. Between tests of EPSP amplitude recorded during the DOWN state, both before and after the pairing, we tested the stability of input and series resistance. If these measures deviated more than ±15%, or if the membrane potential changed more than 8 mV, we discarded the trial. If we did not record at least seven UP states of the course of the pairing epoch, the data set was discarded. Correlation analysis Correlation and partial correlation analysis were performed in MATLAB (corrcoef.m, partialcorr.m). For each neuron, the depolarization traces preceding each pairing on a confirmed circuit reactivation were isolated. These traces were ten point median filtered (10 kHz sampling) and an average binned trace was obtained using 5 ms bins for the preceding 100 ms creating an array for neuron i in time bin t . Correlation analysis was then performed for each time bin between all n neurons’ depolarization and the per cent change in plasticity. For partial correlation, the average depolarization across the entire 100 ms period was obtained, and correlated with plasticity as in equation (4) to get . The partial correlation was performed using a built-in MATLAB function, which, for a single condition, can be formulated as Similar analysis was performed by conditioning with and . Network model We created a spiking neuron network wherein we embedded a Hebbian assembly phase sequence in a recurrent default network of 1,800 neurons. A default recurrent connectivity of 15% was set between randomly connected excitatory neurons. Connectivity from excitatory to inhibitory neurons was 25% and from inhibitory to excitatory neurons was 27%. Synapses were given random axonal conductance delays between 1 and 5 ms. EPSPs were conductance-based and followed discrete exponential decay (excitatory τ =10 ms; inhibitory τ =3.3 ms). Individual assemblies were defined by taking subsets of 100 excitatory neurons and increasing their connectivity to 60%, with a 36% chance for reciprocal connections. We assigned the assemblies an order and added feed-forward connections between 25% of the neurons to generate an assembly phase sequence. A phase sequence was initiated by providing a starting input of randomized PSPs into the first assembly in the sequence for 20 ms. We observed the activity profile of each assembly using a smoothed peristimulus response. In any give sequence, we considered an assembly to have been successfully activated if more than ten neurons spiked in a 5-ms bin. Two plasticity rules were used: a simple STDP rule or a depolarization-dependent CDP rule added to the simple STDP rule. For both rules, we used τ =7.5 ms and Δ w =8.3 × 10 −6 g. For STDP, m =0; for CDP, delay=25 ms, θ =7 mV and m =0.3. A larger m or smaller θ led to a quicker increase in the transition probability P ( X i | X i −1 ). We ran a number of simulations and calculated the probability that an assembly was active given the previous assembly. How to cite this article: Kruskal, P. B. et al . Circuit reactivation dynamically regulates synaptic plasticity in neocortex. Nat. Commun. 4:2574 doi: 10.1038/ncomms3574 (2013).